Retinoic acid receptor alpha is associated with tamoxifen resistance in breast cancer About one-third of oestrogen receptor alpha-positive breast cancer patients treated with tamoxifen relapse. Here we identify the nuclear receptor retinoic acid receptor alpha as a marker of tamoxifen resistance. Using quantitative mass spectrometry-based proteomics, we show that retinoic acid receptor alpha protein networks and levels differ in a tamoxifen-sensitive (MCF7) and a tamoxifen-resistant (LCC2) cell line. High intratumoural retinoic acid receptor alpha protein levels also correlate with reduced relapse-free survival in oestrogen receptor alpha-positive breast cancer patients treated with adjuvant tamoxifen solely. A similar retinoic acid receptor alpha expression pattern is seen in a comparable independent patient cohort. An oestrogen receptor alpha and retinoic acid receptor alpha ligand screening reveals that tamoxifen-resistant LCC2 cells have increased sensitivity to retinoic acid receptor alpha ligands and are less sensitive to oestrogen receptor alpha ligands compared with MCF7 cells. Our data indicate that retinoic acid receptor alpha may be a novel therapeutic target and a predictive factor for oestrogen receptor alpha-positive breast cancer patients treated with adjuvant tamoxifen. Breast cancer (BC) is the most common form of cancer among females, and one out of nine women in western countries will develop BC during their lifetime. The sex hormone oestrogen is central to normal female development and reproductive physiology, but increased and prolonged exposure to oestrogen increases the risk of developing BC [1] . About 80% of BC patients have oestrogen receptor alpha (ER)-positive tumours, making them eligible to adjuvant endocrine treatment, which during more than three decades mainly has consisted of the anti-oestrogen/selective ER modulator tamoxifen. Although tamoxifen treatment reduce recurrence rate by approximately 50%, one-third of the patients receiving adjuvant tamoxifen will be diagnosed with a relapse within 15 years of follow-up, representing up to 25% of all BC patients [2] . As this represents a significant clinical problem, a lot of effort has been put into understanding the resistance mechanisms and finding reliable predictive biomarkers for tamoxifen resistance. For a recent review, see Musgroove and Sutherland [3] . Different gene signatures, proteins and pathways have been proposed to mediate and predict tamoxifen resistance. Overexpression and hyperactivation of tyrosine kinase receptors, such as human epidermal growth factor receptor 2 (HER2) and insulin growth factor receptor, as well as downstream signalling involving the phosphoinositide 3 kinase and mitogen-activated protein kinase cascades, have been shown to mediate resistance to tamoxifen [3] . These pathways converge in the nucleus where they are able to modulate ER activity directly by phosphorylation or indirectly by further modulation of ER coregulators [4] . In addition, a panel of BC anti-oestrogen resistance (BCAR) genes have been identified to mediate tamoxifen resistance in cell lines and clinical material [5] , [6] . A recent study identified activated AKT in transgenic BCAR cell lines [7] . In addition, we have previously linked vascular endothelial growth factor (VEGF) to tamoxifen resistance and as a potential predictor for endocrine-treated BC [8] , [9] , [10] . Interestingly, there is evidence of interplay between the retinoic acid receptor alpha (RARA), another member of the nuclear receptor family, and ER [11] , [12] . ER and RARA share genomic binding sites, and their agonists produce opposite responses [11] . There is also evidence for cooperativity between ER and RARA because response to estradiol (E2) was dependent on the presence of RARA [12] . RARA also seems to be of prognostic value by itself or as a signature including RARA-regulated genes [11] , [12] . Retinoic acid (RA) analogs have been successful anti-tumour agents in acute promyelocytic leukaemia and suggested to have preventive effects in BC [13] , [14] . About 8000-14500 ER-binding sites have been identified in MCF7 cells [11] , [12] , highlighting the complexity of ER signalling [11] , [12] . The Omics technologies present themselves as very useful when studying complex signalling and identifying new predictive biomarkers or therapeutic targets [15] . Despite the success of transcriptome profiling in the prognostic and predictive settings [16] , [17] , [18] , this data cannot be directly extrapolated to proteins because of limited correlation between mRNA and protein levels [19] . Protein-level measurements by mass spectrometry (MS)-based proteomics have matured to give robust identification and quantification data [20] . To study protein-level resistance factors in ER-blocking therapy, we use quantitative MS-based proteomics using previously established BC cell lines, parental MCF7 and the 4-hydroxytamoxifen (4-OHT)-resistant MCF7/LCC2 (LCC2) [21] . Analysis of proteomics data reveals a connection between endocrine resistance and RARA. High RARA protein levels correlate significantly with reduced relapse-free survival (RFS) in steroid receptor-positive BC tumours of patients treated with adjuvant tamoxifen solely. Using a small panel of ER and RARA ligands, with proliferation as end point, we show that ER ligands have decreased effects in LCC2 cells, whereas RARA ligands have an increased effect, in comparison with MCF7. Quantitative proteomics link RARA to tamoxifen resistance Tamoxifen-sensitive and -resistant cells, MCF7 and LCC2, respectively, were treated with an active tamoxifen metabolite, 4-OHT, and compared with untreated cells ( Fig. 1a ). Cytosolic and DNA-bound proteome fractions were generated in this study with the aim to enrich active proteome components. Subcellular fractions were cleaved into peptides, isobaric tags for relative and absolute quantification (iTRAQ)-labelled and separated by narrow range, pH 3.5–4.5 immobilized pH gradient—isoelectric focusing (IPG-IEF). IPG-IEF fractions were analysed by nLC-MALDI-TOF/TOF and nLC-Q-TOF, quantifying 830 proteins ( Supplementary Data 1–3 ). Of these, 629 and 201 proteins were identified in the cytosolic and DNA-binding fraction, respectively, of which 72 were found in both fractions. Experimental robustness of peptide IEF fractionation was verified by plotting the predicted pI value for each peptide against its fraction number revealing a good linear correlation for both the cytosolic ( R 2 =0.99; Spearman’s) and the DNA-binding fraction ( R 2 =0.98; Spearman’s) ( Supplementary Fig. S1 ). Gene ontology (GO) annotation analysis of the identified proteins in the cytosolic and the DNA-binding fraction verified an enrichment of cytosolic and nuclei GO terms in respective subcellular fraction ( Supplementary Fig. S2 ). 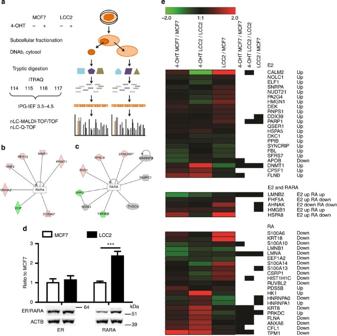Figure 1: Proteomic discovery linking RARA to tamoxifen resistance. (a) Proteomic workflow. The tamoxifen-sensitive MCF7 cell line and the isogenic tamoxifen-resistant cell line LCC2 were treated with 4-OHT for 3 days followed by subcellular fractionation into a DNA-binding (DNAb) and cytosol fraction. Three biological replicates of samples prior and post treatment were digested and iTRAQ-labelled, separated on a narrow-range IPG-IEF strip, pH 3.5–4.5, and analysed by two nLC-MS platforms. (b,c) Ingenuity pathway analysis of changed proteins in the proteomics data indicated a connection of RARA to tamoxifen resistance. (b) Network from comparison of basal levels of MCF7 and LCC2 and (c) changes following 4-OHT treatment in LCC2. Note that ingenuity pathway analysis contains different kinds of data to build connections. For complete networks and explanations, seeSupplementary Fig. S4. * indicates proteins in common withe. (d) Western blot of RARA and ER basal protein levels. (***P<0.001,t-test, values represent mean of two experiments in triplicates±s.e.m.). (e) Connection of RA- and E2-regulated genes to proteins in the DNAb proteomics data set. Heatmap of proteins from the DNAb fraction, separated into E2- and RA-regulated genes based on Huaet al.11,23, respectively. Significantly regulated proteins in this study are highlighted with black boxes to the right of the heatmap. The response to E2 and RA is denoted by up or down. Figure 1: Proteomic discovery linking RARA to tamoxifen resistance. ( a ) Proteomic workflow. The tamoxifen-sensitive MCF7 cell line and the isogenic tamoxifen-resistant cell line LCC2 were treated with 4-OHT for 3 days followed by subcellular fractionation into a DNA-binding (DNAb) and cytosol fraction. Three biological replicates of samples prior and post treatment were digested and iTRAQ-labelled, separated on a narrow-range IPG-IEF strip, pH 3.5–4.5, and analysed by two nLC-MS platforms. ( b , c ) Ingenuity pathway analysis of changed proteins in the proteomics data indicated a connection of RARA to tamoxifen resistance. ( b ) Network from comparison of basal levels of MCF7 and LCC2 and ( c ) changes following 4-OHT treatment in LCC2. Note that ingenuity pathway analysis contains different kinds of data to build connections. For complete networks and explanations, see Supplementary Fig. S4 . * indicates proteins in common with e . ( d ) Western blot of RARA and ER basal protein levels. (*** P <0.001, t -test, values represent mean of two experiments in triplicates±s.e.m.). ( e ) Connection of RA- and E2-regulated genes to proteins in the DNAb proteomics data set. Heatmap of proteins from the DNAb fraction, separated into E2- and RA-regulated genes based on Hua et al . [11] , [23] , respectively. Significantly regulated proteins in this study are highlighted with black boxes to the right of the heatmap. The response to E2 and RA is denoted by up or down. Full size image GO enrichment analysis of downregulated proteins post tamoxifen treatment in the DNA-binding fraction of MCF7 cells showed enrichment of RNA-processing and RNA-splicing GO terms, and upregulated proteins showed an enrichment of GO terms in response to stimulus ( Supplementary Fig. S3 ). In contrast, no GO enrichment could be found by either up- or downregulated proteins in the LCC2 cell line post treatment. We included significantly regulated proteins based on MS proteomics experiment in the pathway and molecular network analysis. These analysis were performed on altered proteins from the three different comparisons, basal level changes between MCF7 and LCC2, and response of MCF7 and LCC2 to 4-OHT. All three comparisons identified p53 as a central network connector ( Fig. 1b and Supplementary Fig. S4A–C ). In addition, RARA was a central network connector in two of the comparisons, comparing basal level changes between LCC2 and MCF7, and 4-OHT treatment of LCC2. No other protein was identified as a central network connector in more than one experimental condition. On the basis of this, and because p53 has been studied in this context by us and others [9] , [22] , we focused on RARA connection to tamoxifen resistance. As an initial evaluation, we performed western blot analysis, which showed higher basal protein levels of RARA in LCC2 than in MCF7, whereas ER levels were similar in both cell lines ( Fig. 1d ). On the basis of the protein network analysis and elevated RARA levels in the resistant cell line, we postulated that RARA-dependent network is involved in tamoxifen resistance. We then studied ER and RARA, mRNA and protein-level changes post treatment with E2, 4-OHT and another ER inhibitor, fulvestrant. MCF7 and LCC2 showed similar ER and RARA protein-level responses to ER ligands ( Supplementary Fig. S5 ). Notably, in the resistant cell line (LCC2), ER and RARA protein and mRNA levels show no correlation post treatment with ER inhibitors (4-OHT and fulvestrant) ( Supplementary Fig. S5 ). Similar to ER, RARA is a nuclear receptor shown not only to antagonize ER function but also to have a cooperative interaction with ER [11] , [12] . This encouraged us to further investigate the role of RARA in tamoxifen resistance. We connected our proteomics data to genes regulated by either E2 or RA and visualized the proteins identified in this study by heatmap ( Fig. 1e and Supplementary Fig. S6 ) (refs 11 , 23 ). Displaying the E2- and RA-regulated proteins separately revealed an increased number of significantly regulated proteins by RA compared with E2 in this study ( Fig. 1e and Supplementary Fig. S6 ). For the cytosolic fraction, there were 23 (8%), 66 (17%) and 29 (7%) significantly regulated proteins that overlapped E2- ,RA- and both E2- and RA-regulated sets, respectively. The corresponding numbers for the DNA-binding fraction were 9 (8%), 23 (17%) and 5 (13%). RARA as a potential predictive marker for adjuvant tamoxifen To test the putative involvement of RARA in tamoxifen resistance concluded from our proteome analysis on the MCF7/LCC2 cell line system, RARA protein levels were analysed on eight breast tumour homogenates ( Fig. 2a ). The tumour lysates were selected from a cohort of tamoxifen-treated patients with a minimum of 15-year follow-up (last inclusion date 31 December 1996). Four patients with early recurrences (<2 years) after primary diagnosis and four patients with a long disease-free follow-up (>7 years) were selected and matched according to age, tumour size and node status ( Supplementary Table S1 ). In this small group, we found that patients with early relapses had higher RARA protein levels than relapse-free patients where low or no expression was observed ( Fig. 2a ). 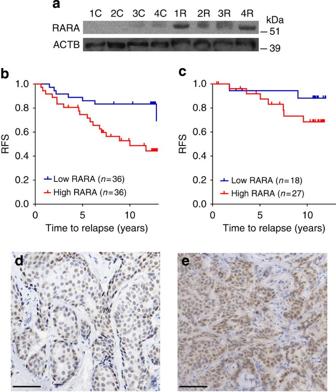Figure 2: High RARA protein levels are correlated with poor outcome in ER-positive BC patients receiving adjuvant tamoxifen. (a) RARA protein-level analysis by western blot on tumour homogenates from four matched pairs of patients. C denotes patients with more than 7 years of disease-free follow-up and R denotes patients with relapse within 2 years. SeeSupplementary Table S1for patient characteristics. (b) RFS for patients in cohort I treated with adjuvant tamoxifen considering their expression of RARA and separated by median value. Determination of RARA was performed on tumour homogenates by ELISA. SeeTable 1for patient characteristics. (c) RFS for patients in cohort II considering their expression of RARA. Determination of RARA was performed by IHC on TMAs. SeeTable 2for patient characteristics. (d,e) Representative images of the IHC scoring of (d) negative and (f) positive samples. In negative cases, there was only weak reactivity in the peripheral parts of tumour strands, whereas in the positive cases, distinct reactivity was seen in the majority of tumour cells. Scale bars, 100 μm. Figure 2: High RARA protein levels are correlated with poor outcome in ER-positive BC patients receiving adjuvant tamoxifen. ( a ) RARA protein-level analysis by western blot on tumour homogenates from four matched pairs of patients. C denotes patients with more than 7 years of disease-free follow-up and R denotes patients with relapse within 2 years. See Supplementary Table S1 for patient characteristics. ( b ) RFS for patients in cohort I treated with adjuvant tamoxifen considering their expression of RARA and separated by median value. Determination of RARA was performed on tumour homogenates by ELISA. See Table 1 for patient characteristics. ( c ) RFS for patients in cohort II considering their expression of RARA. Determination of RARA was performed by IHC on TMAs. See Table 2 for patient characteristics. ( d , e ) Representative images of the IHC scoring of ( d ) negative and ( f ) positive samples. In negative cases, there was only weak reactivity in the peripheral parts of tumour strands, whereas in the positive cases, distinct reactivity was seen in the majority of tumour cells. Scale bars, 100 μm. Full size image The data from western blot analysis encouraged us to further explore the potential value of RARA protein levels using a more quantitative method; hence, we further investigated RARA levels in 72 patients by enzyme-linked immunosorbent assay (ELISA), denoted as cohort 1 ( Table 1 ). Using the median levels of RARA protein as cut-off point, high RARA was found to be significantly correlated with shorter RFS ( P =0.0034, Mantel Cox test) ( Fig. 2b ). Moreover, RARA protein level was the only factor that remained statistically significant for RFS in a Cox proportional multivariate analysis (hazard ratio (HR)=4.1; 95% confidence interval 1.55–11.0; P =0.0046, multivariate Cox proportional hazards) where tumour size (HR=1.2; 95% CI 0.5–2.84), nodal status (HR=1.3; 95% CI 0.56–3.22) and age (HR=1.0; 95% CI 0.96–1.04) also were included but failed to give further information. The wide confidence intervals are explained by the few events in the model. Table 1 Clinicopathological characteristics of patients in validation cohort I. Full size table To see if these findings were consistent with a different analysis platform and patient cohort, we used immunohistochemistry (IHC) to analyse RARA expression on 45 paraffin-embedded tumour tissues on tissue microarrays (TMAs), denoted as cohort II ( Fig. 2c , Table 2 ). The majority of tumours included in the TMA had a high percentage of cells expressing RARA (90–100% of cells) classified as 3+ ( n =27/45). No expression was observed in the stromal compartment of the samples. Representative staining of tumours classified as negative and positive are shown in Fig. 2d , and the cell type specificity of staining is shown in Supplementary Fig. S7 . Expression of RARA did not correlate with tumour size, nodal status, ER, progesterone receptor, histological type, histological grade, HER2 or VEGF. A similar trend to ELISA analysis was seen in this smaller cohort where patients with higher RARA expression exhibited more relapses than patients with low RARA ( P =0.174, Mantel Cox test); 7 out of 27 (26%) compared with 2 out of 18 (11%), respectively ( Fig. 2c ). Table 2 Clinicopathological characteristics of the patients in validation cohort II. Full size table To further understand the characteristics of RARA as a potential predictive marker for tamoxifen treatment, we separated the survival analysis into patients with short follow-up time (0–4 year group), covering drug treatment and drug-overhang period and patients with longer follow-up time post treatment (>4 years group) ( Supplementary Fig. S8 ). In the 0–4-year group, RARA is not a predictive marker ( Supplementary Fig. S8A,C ). In cohort I where RARA was quantified by ELISA, the >4-year group with low RARA patients had significantly better RFS than the high RARA group ( P =0.0028, Mantel Cox test) ( Supplementary Fig. S8B ). The same trend was observed in cohort II measured by IHC ( Supplementary Fig. S8D ). To see how the protein-level measurements correlate with mRNA levels in tumour material, we prepared mRNA and protein from the same pieces of fresh frozen tumours. We observed no correlation between RARA mRNA and protein levels, but a weak correlation for ER is seen ( R 2 =0.37, Spearman’s) ( Supplementary Fig. S9A,B ). In addition, we observed similar basal RARA mRNA levels in MCF7 and LCC2, whereas protein levels were higher in LCC2. For ER, basal mRNA and protein levels were similar between the two cell lines ( Supplementary Fig. S9C,D ). Different response of MCF7 and LCC2 to ER and RARA ligands On the basis of the finding in the cell line material on RARA involvement in tamoxifen resistance and of potential predictive value in clinical material, we again turned to the cell line model to study the functional consequences of perturbing the system. Downregulation of RARA and ER by small interfering RNA (siRNA) decreased proliferation (measured by BrdU incorporation) in both MCF7 and LCC2 to about 70% and 30% of control siRNA for RARA and ER, respectively ( Fig. 3a ). Similar trend, but less pronounced decrease, was observed by measuring cell growth (protein amounts) after siRNA treatment ( Supplementary Fig. S10 ). Both cell lines were growth-limited by p53, used as a positive control ( Fig. 3a ). Downregulation of RARA and ER by siRNA for the proliferation assay was verified by western blot ( Fig. 3b and Supplementary Fig. S11 ). 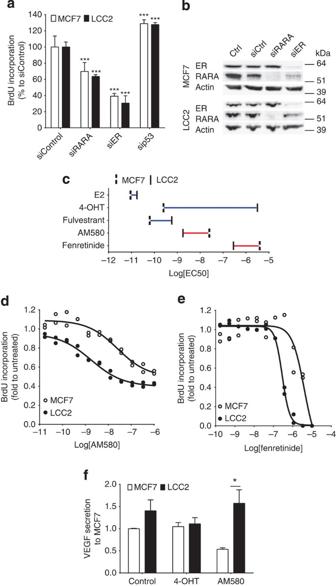Figure 3: Different responses to ER and RARA ligands between tamoxifen-sensitive MCF7 and -resistant LCC2 cell lines. (a) Proliferation of MCF7 and LCC2, measured by percentage of BrdU incorporation after 4 days of culture experiment post 10 nM siRNA transfection. p53 siRNA was included as positive control (***P<0.001, analysis of variance, Dunnett’s test,n=6, ±s.e.m.). (b) Verification of siRNA downregulation experiment of ER and RARA by western blot after 3 days of treatment. (c) EC50 of ER and RARA ligands from dose-response measurements of BrdU incorporation as indande. E2 is the natural ligand of ER, 4-OHT is a tamoxifen metabolite-inhibiting ER, fulvestrant (ICI182780) is an ER antagonist leading to ER degradation, AM580 is a selective RARA agonist and fenretinide is an atypical retinoid. Blue line indicates lower EC50 in MCF7 than LCC2 and red line vice versa. (d,e) Dose-response curves of AM580 and Fenretinide, respectively. Percentage of BrdU-incorporating cells was assessed by IN Cell Analyzer 2000 foraandc–e. (f) Effect on RARA transcribed known resistance factor VEGF by AM580. VEGF secreted into the medium was measured after 3 days treatment with 1 μM 4-OHT or 100 nM AM580. (*P<0.05,t-test, values represent mean of three experiments in triplicates±s.e.m.). Figure 3: Different responses to ER and RARA ligands between tamoxifen-sensitive MCF7 and -resistant LCC2 cell lines. ( a ) Proliferation of MCF7 and LCC2, measured by percentage of BrdU incorporation after 4 days of culture experiment post 10 nM siRNA transfection. p53 siRNA was included as positive control (*** P <0.001, analysis of variance, Dunnett’s test, n =6, ±s.e.m.). ( b ) Verification of siRNA downregulation experiment of ER and RARA by western blot after 3 days of treatment. ( c ) EC50 of ER and RARA ligands from dose-response measurements of BrdU incorporation as in d and e . E2 is the natural ligand of ER, 4-OHT is a tamoxifen metabolite-inhibiting ER, fulvestrant (ICI182780) is an ER antagonist leading to ER degradation, AM580 is a selective RARA agonist and fenretinide is an atypical retinoid. Blue line indicates lower EC50 in MCF7 than LCC2 and red line vice versa. ( d , e ) Dose-response curves of AM580 and Fenretinide, respectively. Percentage of BrdU-incorporating cells was assessed by IN Cell Analyzer 2000 for a and c – e . ( f ) Effect on RARA transcribed known resistance factor VEGF by AM580. VEGF secreted into the medium was measured after 3 days treatment with 1 μM 4-OHT or 100 nM AM580. (* P <0.05, t -test, values represent mean of three experiments in triplicates±s.e.m.). Full size image Further, we studied the response of tamoxifen-sensitive and -resistant cells to ER and RARA ligands (E2, 4-OHT, fulvestrant, AM580, BMS 195 614 and BMS 204 493). MCF7 and LCC2 displayed different dose responses to ER and RARA ligands ( Fig. 3c–e and Supplementary Fig. S12 ). LCC2 was more sensitive to RARA ligands and less sensitive to ER ligands than the parental cell line MCF7 ( Fig. 3c ). Although having approximately the same E2 EC50, MCF7 showed a 1.8-fold increase in proliferation, whereas LCC2 showed a 1.2-fold increase ( Fig. 3c and Supplementary Fig. S12A ). As expected, LCC2 is more resistant to growth inhibition by ER-targeting drugs, compared with MCF7, and does not respond to 4-OHT up to 1 μM, whereas MCF7 responds already at nanomolar concentrations ( Supplementary Fig. S12B ). Interestingly, fulvestrant inhibit proliferation in LCC2, but at higher concentration than in MCF7 ( Fig. 3c and Supplementary Fig. S12C ). The RARA-specific agonist AM580 and the atypical retinoid fenretinide both showed effect at lower concentrations in LCC2 than in MCF7 ( Fig. 3c–e ). The neutral antagonist BMS 195 614 and the inverse agonist BMS 204 493 did not exert any effect on proliferation as measured by BrdU incorporation ( Supplementary Fig. S12D,E ). We have previously reported that VEGF is a tamoxifen-resistance factor in primary BC and that the autocrine VEGF/VEGFR2 loop contributes to LCC2 tamoxifen-resistance phenotype [8] , [10] . VEGF is a known RARA-regulated gene [11] , [24] ; hence, we wanted to study the effect of RARA ligand on VEGF secretion between the cell lines. After 3 days of 4-OHT exposure, secreted VEGF levels in LCC2 seemed to decrease, reaching similar levels to that of treated MCF7 cells. However, a clear difference between cell lines was obtained by treatment with 100 nM of the RARA-specific agonist AM580, which reduced VEGF secretion in MCF7 while increasing it in LCC2 cells ( Fig. 3f ). Fulvestrant changes the proteome in tamoxifen resistance As fulvestrant is an approved drug to treat BC patients, and because both siRNA against ER and fulvestrant treatment leading to ER degradation decreased proliferation in LCC2, we investigated the proteome changes following treatment of fulvestrant compared with non-treated and 4-OHT-treated MCF7 and LCC2 cells. We identified 8,424 protein (1% false discovery rate (FDR)) in two iTRAQ experiments, and after filtering using cut-off set by vehicle replicate consistency and for proteins overlapping the two iTRAQ experiments, 6,470 proteins with quantification values were used for further analysis ( Supplementary Data 4 ). Replicate consistency is shown in Supplementary Fig. S13 . Treatment with 4-OHT induced large proteome changes in MCF7, which were not observed in LCC2 ( Fig. 4a ). On the contrary, fulvestrant induced large proteome changes in both MCF7 and LCC2 with large number of correlating proteins ( Fig. 4b ). In MCF7, fulvestrant- and 4-OHT-changed proteomes showed a similar pattern ( Fig. 4c ). On the other hand, 4-OHT treatment leads to minor proteome changes compared with fulvestrant in LCC2 ( Fig. 4d ). 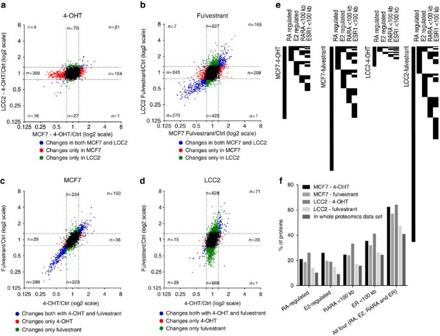Figure 4: Proteome changes in MCF7 and LCC2 cell lines following 4-OHT and fulvestrant treatment. Proteome changes in LCC2 and MCF7 to (a) 4-OHT and (b) fulvestrant showing overlapping set of 6,470 quantified proteins. Similarly, proteome changes in (c) MCF7 and (d) LCC2 to 4-OHT and fulvestrant. Cells were treated with vehicle, 10 nM of 4-OHT or fulvestrant for 3 days, and whole-cell lysates were analysed. Values are the mean of duplicates, and the numbers (n=) denote the number of changed proteins (seeSupplementary Fig. S13for replicate consistency). (e) Connection of changed proteins by 4-OHT and fulvestrant in MCF7 and LCC2 to E2- and RA-regulated genes, and to ER- and RARA-binding sites. (f) Percentage of the changed proteins following 4-OHT and fulvestrant treatment, or the whole data set, which are E2- and RA-regulated or have ER- and RARA-binding sites in genomic proximity. Figure 4: Proteome changes in MCF7 and LCC2 cell lines following 4-OHT and fulvestrant treatment. Proteome changes in LCC2 and MCF7 to ( a ) 4-OHT and ( b ) fulvestrant showing overlapping set of 6,470 quantified proteins. Similarly, proteome changes in ( c ) MCF7 and ( d ) LCC2 to 4-OHT and fulvestrant. Cells were treated with vehicle, 10 nM of 4-OHT or fulvestrant for 3 days, and whole-cell lysates were analysed. Values are the mean of duplicates, and the numbers ( n =) denote the number of changed proteins (see Supplementary Fig. S13 for replicate consistency). ( e ) Connection of changed proteins by 4-OHT and fulvestrant in MCF7 and LCC2 to E2- and RA-regulated genes, and to ER- and RARA-binding sites. ( f ) Percentage of the changed proteins following 4-OHT and fulvestrant treatment, or the whole data set, which are E2- and RA-regulated or have ER- and RARA-binding sites in genomic proximity. Full size image We also looked for connections to ER- and RARA-associated gene sets in the significantly altered proteome part by comparing with E2- and RA-regulated genes and genomic ER- and RARA-binding sites. The proteome changes induced by fulvestrant and 4-OHT all showed overlap with E2- and RA-regulated genes and RARA- and ER-binding sites, which were higher than for the whole proteomics data set ( Fig. 4e ). Biofunctions and canonical pathway analysis in ingenuity pathway analysis identified different cell cycle components as changed, following 4-OHT and fulvestrant treatments, in addition to canonical pathways as aryl hydrocarbon receptor signalling and E2-mediated S-phase entry ( Supplementary Figs S14 and S15 ). The changed proteome following 4-OHT and fulvestrant also show ingenuity pathway analysis connections to both ER and RARA ( Supplementary Fig. S16 ). Tamoxifen resistance changes ER and RARA protein interactors As both MCF7 and LCC2 showed similar dependence on ER and RARA for proliferation, but differences in the response to ligands, we hypothesize that the protein-interaction environment is changed between the cell lines. Experimentally, verified protein–protein interactions to ER and RARA were compiled from Protein Interaction Network Analysis (PINA), Agile Protein Interaction DataAnalyzer (APID) and ingenuity answers databases. Proteins with at least one significant protein ratio between samples ( P -value <0.01, t -test) were used to overlay the quantitative proteomics data for the DNA-binding and cytosol fractions ( Fig. 5a ). Many of the components in the network show differences between the cell lines and treatments. In addition, we analysed the ER- and RARA-connected proteome in relation to fulvestrant and 4-OHT treatment in MCF7 and LCC2. The significantly altered proteins and their relative levels in MCF7 and LCC2 post treatment are visualized in Supplementary Fig. S15 . Altogether, altered levels and patterns of regulation during tamoxifen treatment between MCF7 and LCC2 indicate an altered protein-interaction environment. 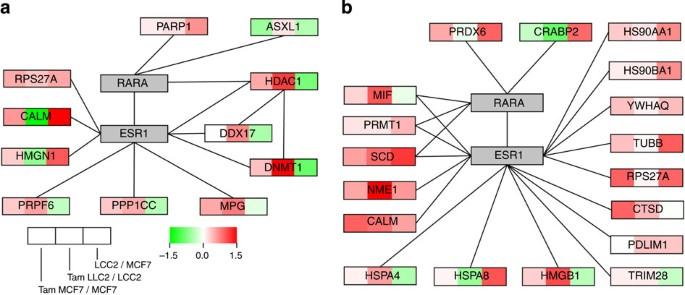Figure 5: Protein–protein interaction network. Network is built with quantitative proteomics data from (a) DNA-binding and (b) cytosolic fraction and indicates an altered protein–protein interaction environment for RARA and ER in tamoxifen resistance. Previously reported protein–protein interactions for ER or RARA were compiled from APID, PINA and ingenuity answers databases and overlaid with quantitative proteomics data from this study. Proteins with at least one significant protein ratio between samples (P-value <0.01,t-test) are displayed. Figure 5: Protein–protein interaction network. Network is built with quantitative proteomics data from ( a ) DNA-binding and ( b ) cytosolic fraction and indicates an altered protein–protein interaction environment for RARA and ER in tamoxifen resistance. Previously reported protein–protein interactions for ER or RARA were compiled from APID, PINA and ingenuity answers databases and overlaid with quantitative proteomics data from this study. Proteins with at least one significant protein ratio between samples ( P -value <0.01, t -test) are displayed. Full size image To gain understanding of tamoxifen-resistant mechanisms and identify predictive markers, we performed quantitative proteomics of a tamoxifen-sensitive and -resistant cell line, MCF7 and LCC2, respectively. Pathway analysis on quantitative proteomics data showed a connection to RARA, which was also manifested when comparing our proteomics data with E2- and RA-regulated genes ( Figs 1 and 4e ). On the basis of these results in cell lines, we used western blot, ELISA and IHC and found that high intratumoural RARA levels, in two small independent cohorts, were correlated with shorter RFS in ER-positive BC patients who received adjuvant tamoxifen treatment ( Fig. 2 ). The two cohorts were primary early-stage ER+BC-treated with adjuvant tamoxifen solely to exclude possible influence of other systemic treatments as chemotherapy, and both cohorts have a median follow-up exceeding 10 years. The negative impact of high RARA levels on patient outcome was not correlated with HER2 positivity. Despite the small patient population, RARA retained as an independent biomarker in a Cox multivariate analysis showing an increased risk for relapse in patients with high RARA of 4.1 times compared with patients with low RARA. However, RARA is not a predictive marker during the drug treatment and drug-overhang period ( Supplementary Fig. S8A,C ), which suggest that there are additional/other resistant mechanisms in this period, for example, the BCAR genes [5] , [7] , [25] . Interestingly, after the drug treatment and drug-overhang period, the predictive potential of RARA is increased compared with entire cohort ( Fig. 2b and Supplementary Fig. S8B,D ). The coupling between RA and senescence has been reported recently [26] , [27] , and high RARA could contribute to senescence phenotype and tumour cell survival during hormonal treatment. A drawback in the relapse analysis is the population size, with consequently few events for statistical analyses. The potential negative impact of high RARA on tamoxifen-resistant BC will be investigated in larger patient populations to elucidate if RARA levels could guide patient selection for longer tamoxifen treatment. The relation between ER and RARA is controversial. First, ER and RARs were described to share many binding regions in the genome, and at these locations, they antagonize each other’s gene expression [11] . In the gene locations studied, ER and RAR were competing for binding to the same element or nearby cis -regulatory elements. In a later study, RARA was shown to be part of the ER transcriptional complex and required for oestrogen-mediated gene expression [12] . In the later study by Ross-Innes et al . [12] , they also concluded that RARA binding to chromatin was dependent on ER. A hypothesis put forth was that RARA might have two roles: one as classic heterodimeric partner to RXR and one as ER-associated protein required to maintain cofactors for ER. As seen in Fig. 3c–e , it is possible that a shift to ER-associated state can provide not only resistance to tamoxifen but also more sensitivity to RARA ligands upon activation. This line of reasoning may also explain that high protein levels predict poor outcome ( Fig. 2 ). In addition, recruitment of nuclear receptors and coregulators requires promotor clearance by ubiquitinylation and proteosomal degradation for gene regulation [28] and treatment of MCF7 with RA-induced degradation of RARA protein without mRNA-level changes [29] . The clearance of active RARA protein may explain why high RARA RNA expression levels predicted positive outcome for 263 patients treated with hormonal therapy [12] . Here we studied correlation of RARA and ER mRNA and protein levels in the cell line model and tumours and detected weak correlation between ER mRNA and protein levels but no correlation between RARA mRNA and protein levels. This indicates that protein-level studies are warranted to study clinical role of RARA levels ( Supplementary Fig. S9 ). In addition, RARA has been shown to epigenetically regulate transcription without the need of ligand [30] , which can be one way to mediate tamoxifen resistance. The complex relationship between ER and RARA and the connection to drug resistance calls for future studies, especially further elucidating protein-level events in model systems and patients. Both cell lines, MCF7 and LCC2, display dependence on ER and RARA for proliferation as shown by siRNA depletion ( Fig. 3a ). However, the response to the small molecule ligands of ER and RARA differ. MCF7 respond at lower concentration to both ER agonist and antagonist ligands compared with LCC2, whereas RARA agonist ligand treatment inhibited cell proliferation in 10-fold lower concentration in LCC2 compared with parental MCF7 ( Fig. 3c–e and Supplementary Fig. S12 ). A plausible explanation is that the protein interactome around ER and RARA has changed as a consequence of acquired tamoxifen resistance ( Fig. 5 ), as competition between coregulators to ER can determine response to tamoxifen [31] . The altered landscape on ER- and RARA-connected proteome was also seen in comprehensive analysis of protein-level changes upon treatment with 4-OHT and fulvestrant comparing MCF7 and LCC2 ( Fig. 4 and Supplementary Fig. S16 ). To monitor the proliferation response of RARA ligands in MCF7 and LCC2, we used an agonist, AM580 (ref. 11 ), a neutral antagonist to RARA, BMS 195 614 and an inverse agonist, BMS 204 493 (ref. 32 ). Surprisingly, BMS 195 614 and BMS 204 493 did not give any proliferation benefit ( Supplementary Fig. S12D,E ), suggesting that there was no agonist pressure in our experimental system, or that RARA functions as cooperative cofactor with ER, apart from its classical transcription factor role. This mode of action is supported by siRNA experiments showing that growth of the resistant cell line is dependent both on RARA and ER ( Fig. 3a ), as well as by the fact that ER-degrading drug fulvestrant have clear effect on resistant cell line ( Figs 3c and 4b and Supplementary Fig. S12C ). The difference in response to AM580 between MCF7 and LCC2 could be explained by an increased dependence of LCC2 on cooperative function of RARA and/or ligand-independent epigenetic transcriptional regulation, and upon AM580 binding, RARA recruits coregulators and inhibits proliferation. Interestingly, AM580 decreased tumour incidence and growth in mouse neu- and wnt1-induced mammary oncogenesis models [33] . Connections to previously known tamoxifen-resistant factors are revealed in the ER and RARA protein-interaction network analysis ( Fig. 5a ) where HDAC1 and DNMT1 are upregulated in LCC2 after 4-OHT treatment. HDAC inhibitors alone have been shown to inhibit growth of sensitive and 4-OHT-resistant MCF7 cells [34] , and in combination with DNMT inhibitors to re-establish ER expression and restore sensitivity to 4-OHT in ER-negative BC cells leading to tumour-growth inhibition [35] . We have previously shown that tamoxifen resistance is associated with increased expression of VEGF and VEGFR2 in primary BC tumours [8] and LCC2 cells [10] . The RA-regulated gene [11] , [24] VEGF and its secretion are modulated differently by RARA ligand AM580 between MCF7 and LCC2 cells ( Fig. 3f ), indicating that RARA response to an agonist ligand has been rewired to increase VEGF secretion in the tamoxifen-resistant setting. As in proliferation assay, the ligand binding to RARA changes the outcome in this case in RA-regulated VEGF expression between MCF7 and LCC2. The pure anti-oestrogen fulvestrant was developed as an alternative to tamoxifen but has in direct comparisons not been found superior to neither tamoxifen nor the later developed aromatase inhibitors. The optimal use of fulvestrant in clinical practice among endocrine therapies is not clear [36] . As LCC2 have higher basal levels of RARA than MCF7, respond to fulvestrant treatment ( Figs 3c and 4b ) and RARA levels were regulated by ER ( Fig. 3b and Supplementary Fig. S7 ), the ER-degrading antagonist fulvestrant may be used to mimic this effect, potentially lowering RARA levels in patients with high RARA. Use of fulvestrant as an alternative to tamoxifen has been suggested before when comparing a tamoxifen-sensitive and -resistant clones of MCF7 (ref. 37 ). Clinical trials with the RA analog fenretinide (retinamide) have shown a decreased risk of second BC [38] and a potential beneficial BC-preventive effect in premenopausal women [14] . The use of retinoids in clinical trials have recently been reviewed (see Connolly et al . [39] ). However, no RARA-selective compound has been tested for treatment of endocrine-resistant BC. In our pre-clinical model, LCC2 are more sensitive than MCF7 to inhibition of proliferation by RARA ligand fenretinide ( Fig. 3d ), suggesting an alternative treatment of patients with tamoxifen resistance or high RARA expression. In conclusion, our quantitative proteomics discovery in BC cell lines and validation in two independent patient cohorts implicate RARA in tamoxifen resistance and constitute a potential predictive marker for ER+BC as well as a potential drug target. Proteomics of DNA-binding and cytosol subcellular fractions For proteomics experiments, MCF7 and LCC2 cells were treated with 1 μM 4-OHT for 3 days and fractionated into a cytosolic and DNA-binding fraction (Q proteome nuclear kit; Qiagen). Three biological replicates of each sample were labelled with iTRAQ 4plex according to the manufacturer’s protocol (Applied Biosystems, Framingham, MA, USA) and separated by IPG-IEF on a narrow range pH 3.5–4.5 strip (GE Healthcare) as described previously [40] . Extracted fractions from the IPG-IEF were separated using an Ultimate 3000 LC system (Dionex/LC Packings, Sunnyvale, CA, USA) coupled to a Probot MALDI spotting device and then analysed on an 4800 MALDI-TOF/TOF instrument (Applied Biosystems). Fractions were also analysed using an Agilent 1200 nano-LC system coupled to an Agilent 6530 Q-TOF via a Chip-Cube. Protein pilot and spectrum mill were used to match the spectra. Protein identification were limited to a FDR of <1%. Protein quantification and peptide quality control (PQPQ) was used for quantification of replicates [41] . Ligands and siRNA Ligands, fulvestrant (ICI 182780), AM580, BMS 195 614, BMS 493 (BMS 204 493) and fenretinide were from Tocris Biosciences. E2 and 4-OHT were purchased from Sigma. Ligands were dissolved in dimethylsulphoxide and three-fold dilution series over 11 points were done by Echo 550 liquid handler. Cells were treated with ligands for 3 days and final dimethylsulphoxide concentration was <0.1% for all concentrations. Replicates for the same ligand concentration were on different Costar black clear bottom 96-well plates. siRNA on-targetplus smartpool targeting RARA (L-003437-00), ESR1 (L-003401-00), p53 (L-003329-00) and non-target (D-001810-01) were from Dharmacon and reverse transfected using RNAiMax (Invitrogen). For siRNA, treatments were done for 4 days using 10 nM siRNA. Proliferation Cells were stained using GE Healthcare Cell Proliferation Fluorescence kit and Hoechst 33342 (Sigma). Images were collected using an IN Cell Analyzer 2000 acquiring four images per well with a Nikon × 10/0.45 objective. Fluorescence was monitored using excitation and emission filters, respectively, of: (1) 350/50 and 455/50 nm for Hoechst 33342 and (2) 645/30 and 705/72 nm for Cy5, Quad 2 polychroic and hardware laser autofocus. Images were analysed with IN Cell Analyzer Workstation 3.7 software using the Multi Target Analysis module. Segmentation, nuclei (Hoechst) was defined using top-hat and Colditz [1] (Cy5) using pseudo from nuclei, minimum area 50 μm 2 . The proportion of proliferating cells, positive for both Hoechst 33342 and Cy5 signal, was determined using a decision tree filter. Patient cohorts The study design was done according to the REMARK criteria for tumour marker studies [42] and approved by the research ethical boards of Linköping University and the Karolinska Institutet, Stockholm, Sweden. Two independent patient cohorts were used for validation studies. Both included patients with ER and/or PR positive tumours of primary early-BC stage I–III having received tamoxifen as the sole systemic adjuvant therapy and have previously been subjects for extensive research, leaving fewer patients for analyses of RARA. Patient cohort I originally consisted of 449 patients diagnosed from 1991 to 1996 in the south east health-care region of Sweden. This patient population and sample preparation have previously been described in detail and used for determination of intratumoural VEGF content [43] and other markers, not yet published, which reduced the available material to 72 patients tumour homogenates. Determination of RARA levels in this cohort was done by western blot ( n =8) and use of a commercial ELISA (USCN cat no. E90976Hu) ( n =72). The pilot verification included tumour homogenates from four patients who relapsed within 2 years of tamoxifen treatment (denoted relapse) and four patients with a disease-free follow-up time of more than 7 years to circumventing a possible ‘hangover’ effect of tamoxifen (denoted control). Patients were matched into four pairs defined by age, tumour size and node status ( Supplementary Table S1 ). Patients in cohort II were diagnosed from 1993 to 1996 at two institutions in Stockholm, Sweden. The original cohort includes tumour homogenates from 404 patients and which has been described in detail elsewhere where data on histological grade and HER2 also are found [44] . The TMA used in this study consisted of 45 available paraffin-embedded tumours. Basal clinical and BC-marker features for the two cohorts are shown in Tables 1 and 2 . Construction of TMAs A TMA was constructed from formalin-fixed primary tumours ( n =95). Before TMA construction, all tumours were evaluated by an experienced pathologist by staining with hematoxylin. Two cores were taken from donor block areas morphologically representative of the tumour and used for the construction of the recipient TMA blocks. This was done using a Beecher Manual Arrayer 1 (Beecher Instruments, Silver Spring, MD, USA) with a punch diameter of 1 mm. From the TMA, 4-μM paraffin sections were sliced and put on glass slides and subsequently dewaxed and rehydrated. The slides were thereafter boiled in citrate buffer (pH 6.0, 12 min at 800 W and 20 min at 250 W), allowed to cool and rinsed with PBS. After blocking in 1% BSA solution, the slides were incubated with RARA (sc-551) as the primary antibody. The staining of RARA was visualized by applying a biotinylated secondary antibody followed by ABC and diaminobenzidine as a chromogene (Vector Laboratories) and counterstained with hematoxylin and eosin. The staining of RARA was evaluated by two trained pathologists in a blinded fashion (A.K. and G.M.). Survival analyses For correlation and survival analyses, patients were operated in two groups; low versus high RARA separated by median value. Pearson’s χ 2 -test was used to analyse possible associations between RARA levels and standard BC parameters including S-phase fraction as well as previously determined VEGF. Factors investigated (RARA, tumour size, lymph-node status, S-phase fraction, VEGF and age) were dichotomized. Data were available on HER2 and histological grade in patient cohort II. HER2 was operated as positive versus negative, and histological grade as grade I and II versus grade III. Survival was estimated using the Kaplan–Meier method, and the comparison between study groups was performed with the log-rank test. The end-point RFS was calculated as time from diagnosis to the first documented recurrence. All tests were two-sided, and P -values <0.05 were considered significant. All calculations were made with SPSS 16.0. Protein expression analysis by western blot After 3 days of treatment, cells were collected and lysed using the radioprecipitation assay buffer (50 mM Tris, pH 7.4, 150 mM NaCl, 0.5% Igepal, 5 mM EDTA and 0.1% SDS) supplemented with Mini protease inhibitor cocktail. Cell lysates and patient tumour homogenates were quantified using the DC Protein Assay Kit (Bio-Rad). A total of 50 μg of cell lysate and 30 μg of tumour homogenate per sample were run on SDS-PAGE gels (NuPage Bis Tris 10%; Invitrogen), blotted and subsequently incubated overnight with ESR1 (Sc-8002, 1:500), RARA (sc-551, 1:500), actin (Sc-1616-R, 1:2,000) from Santa Cruz Biotechnology and GAPDH from Trevigen (2275-PC-100, 1:2,000). After incubation with anti-mouse or anti-rabbit IgG-horseradish peroxidase conjugate (1:5,000) (GE Healthcare), bands were detected using ECL Western Blotting Detection Reagents (Amersham). Quantitative PCR analysis Protein, mRNA and DNA were extracted using the AllPrep DNA/RNA/Protein Mini Kit (Qiagen, Hilden, Germany), and mRNA concentration was measured using NanoDrop (Thermo Fisher Scientific). RNA of 500 ng was retrotranscribed using High Capacity RNA to cDNA kit (Invitrogen) according to the manufacturer’s instructions. cDNA of 10 ng was used for each quantitative PCR reaction, and the reactions were performed in a 96-well plate using TaqMan Gene Expression Assay (Invitrogen). The following assays were used: RARA (Hs00940446_m1) and ESR1 (Hs00174860_m1); for normalization purposes, 18S (Hs99999901_s1) was used. Changes in mRNA levels in the cell lines were calculated with the ΔΔCt method, based on Ct cycle values for the target gene of interest normalized to 18S and then expressed as fold change to the untreated samples. Relative mRNA levels in the tumours were determined using the ΔCt method, only based on Ct cycle values for the target gene of interest normalized to 18S. Assessment of secreted VEGF Conditioned media was collected before cell collection and stored at −20 °C after protein determination. The protein levels of VEGF were measured on conditioned media by a quantitative ELISA kit for human VEGF-A (Quantikine; R&D Systems, Minneapolis, MN, USA) according to the manufacturer’s protocol. Proteomics of 4-OHT- and fulvestrant-treated cells MCF7 and LCC2 cells were treated with 10 nM 4-OHT or fulvestrant for 3 days and then lysed in 4% SDS, 25 mM HEPES and 1 mM dithiothreitol. Cell lysates were heated to 95 °C for 5 min followed by sonication for 1 min and centrifugation at 14,000 g for 15 min. The supernatant was subjected to spin filter sample preparation. The tryptic peptides were iTRAQ-labelled according to the manufacturer’s protocol (Applied Biosystems) and cleaned by a strata-X-C-cartridge (Phenomenex) before separation by IPG-IEF on a pH 3.7–4.9 strip as described above. Before analysis of IPG-IEF fractions on the Thermo Scientific LTQ Orbitrap Velos, peptides were separated using an Agilent 1200 nano-LC system. Samples were trapped on Zorbax 300SB-C18, 5 μm, 5 × 0.3 mm, and separated on a NTCC-360/100-5-153 column (Nikkyo Technos., Ltd) using a gradient of A (3% ACN, 0.1% FA) and B (95% ACN, 0.1% FA), ranging from 3 to 40% B in 90 min with a flow of 0.4 μl min −1 . The LTQ Orbitrap Velos was operated in a data-dependent mode, selecting five precursors for sequential fragmentation by collision-induced dissociation (CID) and higher-energy collisional dissociation (HCD), analysed by the linear iontrap and orbitrap, respectively. Proteome discoverer 1.3 with sequest-percolator was used for protein identification. Spectra were matched to ensembl 68, limited to human protein sequences, and results were filtered to 1% FDR. For detailed methods, see Supplementary Information . Accession codes : The mass spectrometry proteomics data have been deposited to the ProteomeXchange Consortium via the PRIDE partner repository [45] under the accession code PXD000281 . How to cite this article: Johansson, H. J. et al . Retinoic acid receptor alpha is associated with tamoxifen resistance in breast cancer. Nat. Commun. 4:2175 doi: 10.1038/ncomms3175 (2013)